A general strategy for preparing pyrrolic-N4type single-atom catalystsviapre-located isolated atoms Single-atom catalysts (SACs) have been applied in many fields due to their superior catalytic performance. Because of the unique properties of the single-atom-site, using the single atoms as catalysts to synthesize SACs is promising. In this work, we have successfully achieved Co 1 SAC using Pt 1 atoms as catalysts. More importantly, this synthesis strategy can be extended to achieve Fe and Ni SACs as well. X-ray absorption spectroscopy (XAS) results demonstrate that the achieved Fe, Co, and Ni SACs are in a M 1 -pyrrolic N 4 (M= Fe, Co, and Ni) structure. Density functional theory (DFT) studies show that the Co(Cp) 2 dissociation is enhanced by Pt 1 atoms, thus leading to the formation of Co 1 atoms instead of nanoparticles. These SACs are also evaluated under hydrogen evolution reaction (HER) and oxygen evolution reaction (OER), and the nature of active sites under HER are unveiled by the operando XAS studies. These new findings extend the application fields of SACs to catalytic fabrication methodology, which is promising for the rational design of advanced SACs. Single-atom catalysts (SACs) [1] have attracted considerable interest due to their superior catalytic activity and unique selectivity towards different chemical reactions, including CO oxidation [1] , [2] , hydrogenation [3] , dehydrogenation [4] , [5] , and electrochemical reactions [6] , [7] , [8] . Recently, the application of SACs has been widely extended to various research areas [9] , [10] , [11] , [12] , [13] , [14] including energy storage systems like Li-S batteries [15] , enzyme catalysis [16] , photocatalysis [17] , and even cellular NO sensor [18] . Therefore, SACs are continuously showing great potentials for wide applications. The most significant distinction between SACs and other types of catalysts is their unique single-atom-site, which both increases the atom utilization efficiency and tailors the interaction between the reactant and metal atoms through the adsorption and activation process. For example, Yan et al. reported the Pd 1 /graphene SACs showed a high butane selectivity in the hydrogenation of 1,3-butadiene, where the adsorption of 1,3-butadiene on Pd 1 was mainly in a mono-π mode, which differs from that on Pd bulk [3] . Duchesne and co-workers showed that the Pt single atoms on Au nanoparticles (NPs) exhibited superior catalytic performance in formic acid oxidation. Such a high activity of Pt 4 Au 96 is ascribed to the weakened CO adsorption on single and few Pt atoms than that on Pt bulk [19] . Li and co-workers demonstrated that the Pt 1 /Co 3 O 4 exhibited a much weaker H 2 adsorption energy than Pt bulk, thus leading to its high catalytic performance in the dehydrogenation of ammonia borane [5] . However, because of their highly un-saturated coordination environment, heterogeneously supported single atoms possess a dramatically increased surface-free energy, which can lead to their aggregation into NPs, particularly at high metal loadings. Recently, some strategies have been developed to achieve relatively high-loading SACs. These methods include zeolite or mesoporous carbon to stabilize single atoms through a confinement strategy [20] , [21] , [22] , [23] , metal-organic frameworks (MOFs) to achieve SACs through high-temperature pyrolysis [24] , metal NPs to achieve SACs through high-temperature migration [25] , [26] , and a high-temperature shock wave treatment to achieve high loading SACs [27] . However, there are yet some restrictions on these newly developed methods such as general applicability. Therefore, developing a general approach for the synthesis of various types of SACs is highly desired. Atomic layer deposition (ALD), a sequential surface reaction relying on a self-limiting process is used to synthesize non-noble single atoms such as Fe and Co [28] , [29] . Unfortunately, it results in a low metal loading and the formation of NPs, especially on carbon-based supports due to the high dissociation barrier and predominantly physical adsorption of metal precursors [28] , [29] , [30] , [31] . Therefore, a new reasonable route to produce SACs by ALD may be achieved by lowering the dissociation energy of the ALD precursor. For instance, this high dissociation energy might be strongly reduced on a metal surface [31] , [32] , [33] . Accordingly, the use of metal single atoms as the catalyst to facilitate the dissociation of ALD precursors to synthesize SACs would be very promising. To the best of our knowledge, this new SACs producing strategy that uses surface single atoms as the catalysts has never been reported. Moreover, the ALD method is feasible to obtain single atoms on various supports, which not only provides a new way to achieve SACs with dual atomic sites but also extends the application fields of SACs to the catalytic fabrication methodology. In this work, we firstly verified the strategy by using supported Pt single atoms on N-doped carbon nanosheets (Pt 1 /NCNS) as the catalyst to synthesize Co SAC through ALD. X-ray absorption spectroscopy (XAS) results reveal singly dispersed Co 1 atoms. Interestingly, the Pt 1 atoms are still atomically dispersed after Co deposition, as confirmed by XAS and high-angle annular dark-field scanning transmission electron microscopy (HAADF-STEM). Furthermore, we also show that this synthesis strategy is general and can also be easily extended to achieve Fe and Ni SACs. X-ray absorption near edge structure (XANES) simulation and extended X-ray absorption fine structure (EXAFS) analysis results demonstrate that the achieved Co, Fe, and Ni SACs are in a M 1 -pyrrolic-N 4 structure (M=Fe, Co, and Ni). Density functional theory (DFT) calculations show that Pt 1 atoms promote the dissociation of Co(Cp) 2 into CoCp and Cp fragments. The Co(Cp) product further deposited on the substrate through strong chemisorption, thus leading to a higher metal loading and formation of Co 1 atoms. These SACs were evaluated under hydrogen evolution reaction (HER) and the nature of single-atom sites are unveiled by the operando XAS studies. Moreover, in the oxygen evolution reaction (OER), the Ni 1 SAC showed much higher activity than Fe 1 and Co 1 SACs, which is in line with the DFT predictions. Direct fabrication of Pt and Co single atoms on NCNS using ALD Graphene like NCNS (Fig. 1a and Supplementary Fig. 1 ) was firstly achieved using C 3 N 4 as the template and glucose as the carbon source [34] . N K -edge XANES results indicate that there are various types of N species including pyridinic, pyrrolic, and graphitic N on NCNS (Fig. 1b ) [35] . According to the literature, the N defects can coordinate with metal species and form a stable SAC [7] . Therefore, the NCNS substrate shows high potential for the synthesis of SACs. After performing one cycle of Pt ALD on NCNS, well-dispersed Pt single atoms were confirmed by HAADF-STEM (Supplementary Fig. 2 ) and XAS results (Supplementary Fig. 3 ) [36] . The loading of Pt is as high as 2.0 wt% based on the inductively coupled plasma optical emission spectrometer (ICP-OES) results. Fig. 1: Characterizations for pristine NCNS, Co-NPs/NCNS, and proposed synthesis strategies for Co SAC. a HAADF-STEM image of NCNS. b XANES of NCNS at N K edge. c FT-EXAFS of Co-NPs/NCNS, as well as Co foil and Co 3 O 4 reference at Co K edge, respectively. d Assumption of the Co ALD process on pristine NCNS and Pt 1 /NCNS. The white, brown, blue, and orange spheres represent H, C, N, and Co, respectively. Full size image Since the NCNS shows great potential to support Pt 1 atoms, it has the possibility to act as a suitable substrate for other types of SACs. Using ALD, we performed one cycle of Co ALD on NCNS with Co(Cp) 2 and O 2 as the precursors. However, unlike the formation of Pt 1 atoms, we found obvious Co NPs/clusters in HAADF-STEM (Supplementary Fig. 4a ) and Co-Co coordination from the EXAFS results at the Co K edge (Fig. 1c ), indicating the formation of Co NPs (Co-NPs/NCNS). Besides the formation of Co NPs, we also noticed a very low metal loading of Co (0.5 wt%). Such a low loading of Co indicates limited physisorption after the dose of Co(Cp) 2 precursor, and the unreacted Co(Cp) 2 would be purged away by N 2 as illustrated in (Supplementary Fig. 5 ), leading to a low effective Co deposition [30] . Unfortunately, the weak adsorption effect of Co(Cp) 2 on NCNS will form Co NPs due to the weak interaction between Co species and substrate when O 2 is introduced. Therefore, the direct utilization of the Co ALD process to produce Co single atoms on NCNS is not practical. Synthesizing Co, Fe, and Ni SACs using pre-located isolated Pt 1 atoms Inspired by previous research, the dissociation of Co(Cp) 2 will be enhanced on the metal surface [37] . In our system, the Pt single atoms are easy to achieve, and the Pt-based catalysts are active in many chemical reactions. Therefore, the singly dispersed Pt 1 atoms may have a similar ability and are likely capable to decrease the dissociation energy of Co(Cp) 2 , which may increase the Co loading and more importantly to achieve Co single atoms. With this idea in mind, we firstly conducted one cycle of Pt ALD on NCNS to achieve Pt 1 /NCNS and followed up with one cycle of Co ALD to verify our assumption (Fig. 1d ). After performing one cycle of Co ALD on Pt 1 /NCNS substrate, the Co K edge EXAFS of this sample exhibits only one single peak at 1.57 Å (Fig. 2a ), which can be attributed to the first shell of Co-C/N/O coordination. Meanwhile, the coordination of Co-Co is negligible, indicating that the Co species mostly exist as single atoms from the new synthesis strategy. In the following parts, this sample is denoted as Co 1 Pt 1 /NCNS. Fig. 2: XAS characterizations for M 1 Pt 1 /NCNS catalysts. a – c Radial distribution curve from FT-EXAFS of Co-NPs/NCNS, Co 1 Pt 1 /NCNS, Fe-NPs/NCNS, Fe 1 Pt 1 /NCNS, Ni-NPs/NCNS, and Ni 1 Pt 1 /NCNS, respectively, as well as their corresponding foil and oxide reference at Co, Fe, and Ni K edges. d – f Wavelet-transformed spectra of Co 1 Pt 1 /NCNS, Fe 1 Pt 1 /NCNS, Ni 1 Pt 1 /NCNS, as well as their corresponding foil and oxide reference at Co, Fe, and Ni K edges. g and h XANES and FT-EXAFS of Pt 1 /NCNS, Co 1 Pt 1 /NCNS, Fe 1 Pt 1 /NCNS, and Ni 1 Pt 1 /NCNS, respectively, as well as Pt foil and PtO 2 reference at Pt L 3 edge. i ICP-OES results of M (Fe, Co, and Ni) metal loadings. Full size image In order to further extend the application of this synthesis strategy to other SACs such as Fe and Ni, we have chosen to use Fe and Ni ALD precursors with similar chemical structures as that of Co, i.e., ferrocene and nickelocene, respectively. Similarly, Fe and Ni single atoms also cannot be achieved by ALD on pristine NCNS as revealed by Fe-Fe and Ni-Ni coordination in the EXAFS (Fig. 2b, c ) and TEM results (Supplementary Fig. 4 ). In contrast, the Fe-Fe and Ni-Ni coordination are significantly depressed when performing one cycle of Fe and Ni ALD on Pt 1 /NCNS (Fe 1 Pt 1 /NCNS and Ni 1 Pt 1 /NCNS) (Fig. 2b, c ). Wavelet-transform EXAFS results further verified the atomically dispersed Co, Fe, and Ni single atoms, which differs from that of their foil and oxide (Fig. 2d, f ). More interestingly, the Pt L 3 edge XANES (Fig. 2g ) and X-ray Photoelectron Spectroscopy (XPS) (Supplementary Fig. 6 ) results show inconspicuous differences, indicating the electronic properties of Pt on these M 1 Pt 1 /NCNS (M=Fe, Co, and Ni) samples are close to that on Pt 1 /NCNS. Pt L 3 edge EXAFS results further confirm the stable local structure of the Pt 1 atom (Fig. 2h ). Typical EXAFS fitting on Co 1 Pt 1 /NCNS at Pt L 3 edge also demonstrates the unchanged atomic nature of Pt single atoms (Supplementary Fig. 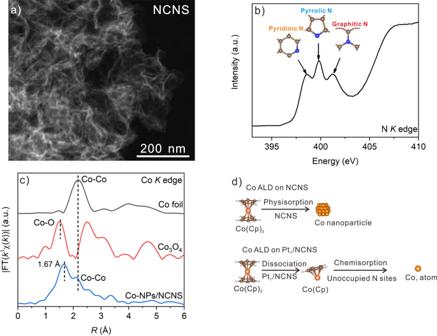Fig. 1: Characterizations for pristine NCNS, Co-NPs/NCNS, and proposed synthesis strategies for Co SAC. aHAADF-STEM image of NCNS.bXANES of NCNS at NKedge.cFT-EXAFS of Co-NPs/NCNS, as well as Co foil and Co3O4reference at CoKedge, respectively.dAssumption of the Co ALD process on pristine NCNS and Pt1/NCNS. The white, brown, blue, and orange spheres represent H, C, N, and Co, respectively. 7 and Supplementary Table 1 ). These results indicate that the Pt 1 atoms are still atomically dispersed after the deposition of Co, Fe, and Ni. This observation provides strong evidence that the Pt 1 atoms only act as the catalyst, while they change the deposition process of Co, Fe, and Ni, but does not lose the atomic dispersion or form a Pt-Co/Fe/Ni cluster, because of the lack of metal-metal coordination in Pt L 3 , Fe, Co, and Ni K edges EXAFS results. Subsequently, we examined the Co loading through ICP-OES after performing one cycle of Co ALD on pristine NCNS and Pt 1 /NCNS (Fig. 2i ). The ICP-OES results show that the Co loading of Co 1 Pt 1 /NCNS (1.8 wt%) is more than three times higher than that of Co-NPs/NCNS (0.5 wt%). Similar results are also observed on Fe and Ni, showing low Fe and Ni loadings on Fe-NPs/NCNS and Ni-NPs/NCNS (0.6 and 0.5 wt%) but much higher on Fe 1 Pt 1 /NCNS and Ni 1 Pt 1 /NCNS (1.6 and 2.2 wt%), respectively. These results unambiguously demonstrate that the Pt 1 atoms change the adsorption model of M precursors to predominantly chemisorption, which promotes the degree of effective deposition. However, when the M ALD was performed on pristine NCNS, physisorption is dominant, thus leading to a low metal loading because of less effective deposition. Morphology of M 1 Pt 1 /NCNS catalysts The morphology of M 1 Pt 1 /NCNS catalysts is characterized by HAADF-STEM. As shown in Fig. 3a, e, i , no observable Pt or M NPs can be found at low magnification. Energy dispersive X-ray (EDX) mapping results show the Pt and M elements are well-dispersed on the NCNS substrate (Fig. 3b, f, j and Supplementary Figs. 8 to 10 ), indicating their uniform dispersion and high density. At high magnification, high-density bright Pt single atoms (white circles) can be found on Co 1 Pt 1 /NCNS (Fig. 3c and Supplementary Fig. 8f ), Fe 1 Pt 1 /NCNS (Fig. 3g and Supplementary Fig. 9f ), and Ni 1 Pt 1 /NCNS (Fig. 3k and Supplementary Fig. 10f ). All the visible Pt atoms are singly dispersed without any obvious clusters or NPs. Meanwhile, some isolated atoms with less brightness (red circles) were also found to reside nearby the bright Pt 1 atoms, which can be assigned to Fe, Co, and Ni single atoms due to their lower Z-contrast. Furthermore, when the electron energy loss spectroscopy (EELS) was measured at the atoms with less brightness on Co 1 Pt 1 /NCNS, the signals of Co L 2 and L 3 could also be detected (Fig. 3d ), confirming the existence of Co 1 atoms. Similar results can be also found on Fe 1 Pt 1 /NCNS (Fig. 3h ) and Ni 1 Pt 1 /NCNS (Fig. 3i ). Based on the HAADF-STEM results, the Fe, Co, and Ni-Pt pairs are absent. Taken together, the EXAFS and HAADF-STEM results demonstrate the single-atom nature of both Pt and M atoms on NCNS. Fig. 3: Morphology of M 1 Pt 1 /NCNS catalysts. HAADF-STEM images of Co 1 Pt 1 /NCNS ( a ), Fe 1 Pt 1 /NCNS ( e ), and Ni 1 Pt 1 /NCNS ( i ) at low resolution and corresponding EDX mapping ( b , f , and j ). HAADF-STEM images on Co 1 Pt 1 /NCNS ( c ), Fe 1 Pt 1 /NCNS ( g ), and Ni 1 Pt 1 /NCNS ( k ) samples. The white circles highlight the Pt single atoms. The red circles highlight the Co, Fe, and Ni single atoms, respectively. d , h , and l Corresponding EELS spectra at the location of red dash circle in c , g , and k . Full size image Structure identification of M SACs Using this synthesis strategy, we have successfully achieved Co, Fe, and Ni SACs. Unveiling the local structure of these SACs is critical to understand the synthesis mechanism and their catalytic applications. XANES spectroscopy is very sensitive to the local geometric structure of the photon-absorbing atom, which provides a better option to understand the local atomic structure. As shown in Fig. 4a to c , the Co 1 Pt 1 /NCNS, Fe 1 Pt 1 /NCNS, and Ni 1 Pt 1 /NCNS at Co, Fe, and Ni K edge XANES spectra, respectively, show significant differences from their corresponding foil and oxide references. We also notice that the XANES spectra of Co 1 Pt 1 /NCNS, Fe 1 Pt 1 /NCNS, and Ni 1 Pt 1 /NCNS are nearly identical, indicating a similar local coordination environment of M 1 Pt 1 /NCNS catalysts. This can be delineated since the k-dependent absorber phase shift of Fe, Co, and Ni, adjacent in the periodic table, is very similar. Taking the first derivative XANES of M 1 Pt 1 /NCNS, the energy position of the point of first inflection suggests that the oxidation states of Fe, Co, and Ni are close to +3, +2, and +2, respectively. These observations are perfectly in line with the XPS results (Supplementary Fig. 11 ). Fig. 4: Identification of the local structure of M 1 Pt 1 /NCNS catalysts. a – c The experimental K -edge XANES spectra and first derivative curves (insets) of M 1 Pt 1 /NCNS and references samples. d – f Comparison between the experimental K -edge XANES spectra of M 1 Pt 1 /NCNS and the simulated spectra. Some of the main features reproduced are highlighted at points “a” to “d”. Fitting results of the k 3 -weighted FT spectrum of M 1 Pt 1 /NCNS at Co ( g ), Fe ( h ), and Ni ( i ) K edges. The white, brown, blue, red, orange, green, and pink spheres represent H, C, N, O, Co, Fe, and Ni, respectively. Full size image Focusing on the Co 1 Pt 1 /NCNS catalyst, we first compared the modeling XANES result based on a recently reported Co-C 4 -O 2 type Co 1 atom on graphene using ALD (Supplementary Fig. 12a ) [38] . Significant differences can be observed between the theoretical simulated XANES and experimental results, indicating the necessity to consider the critical role of N atoms. We then further compared the reported pyridinic-N 4 -based Co 1 -N 4 structure, which still shows the obvious difference with our experimental XANES results (Supplementary Fig. 12b ), suggesting the existence of defects in this model as well. Then we progressively add one and two end-on oxygen moieties along the axial direction of the pyridinic Co 1 -N 4 structure (Supplementary Fig. 12c, d ). Although parts of the experimentally resolved features can be reproduced and achieve a satisfactory agreement with the Co 1 Pt 1 /NCNS Co K edge XANES results, the short Co-N bonding distance (less than 1.90 Å) disagrees with our EXAFS results (Fig. 2a ). Considering that there is a large proportion of pyrrolic-N in the NCNS support, the possibility of a pyrrolic-N 4 type Co 1 -N 4 structure cannot be ruled out. As shown in Supplementary Fig. 12e , the simulated XANES result of pyrrolic-N 4 -based Co 1 -N 4 showed much better conformity than the pyridinic-N 4 structure. We then further added one molecule of dioxygen with end on coordination on Co 1 atom, the features from “b” to “d” are well reproduced but the pre-edge feature “a” is exaggerated (Supplementary Fig. 12f ). However, when we added another molecule of dioxygen on the Co 1 atom at the opposite side, all the features from “a” to “d” can be correctly reproduced (Fig. 4d ). Similarly, the simulated 2O 2 -Fe 1 -pyrrolic N 4 and 2O 2 -Ni 1 -pyrrolic N 4 XANES spectra (Fig. 4e, f ) show the most satisfactory results comparing with other DFT optimized structures (Supplementary Figs. 13 and 14 ). It is important to note, this is the first time that general M 1 -pyrrolic N 4 type SACs can be achieved using ALD, as this type of SACs is usually achieved through high-temperature pyrolysis and ball-milling methods [39] , [40] . Bedsides the above XANES simulation, we also carried out the EXAFS fitting and the results consistently demonstrate the 2O 2 -M 1 -pyrrolic N 4 moiety (Fig. 4g to i , Supplementary Figs. 15 to 18 , and Table 1 ). 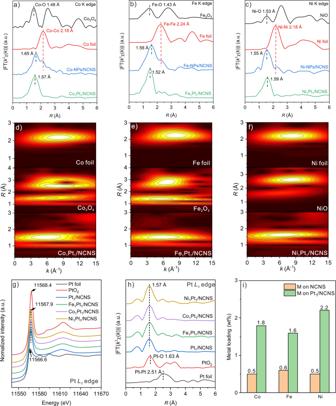Fig. 2: XAS characterizations for M1Pt1/NCNS catalysts. a–cRadial distribution curve from FT-EXAFS of Co-NPs/NCNS, Co1Pt1/NCNS, Fe-NPs/NCNS, Fe1Pt1/NCNS, Ni-NPs/NCNS, and Ni1Pt1/NCNS, respectively, as well as their corresponding foil and oxide reference at Co, Fe, and NiKedges.d–fWavelet-transformed spectra of Co1Pt1/NCNS, Fe1Pt1/NCNS, Ni1Pt1/NCNS, as well as their corresponding foil and oxide reference at Co, Fe, and NiKedges.gandhXANES and FT-EXAFS of Pt1/NCNS, Co1Pt1/NCNS, Fe1Pt1/NCNS, and Ni1Pt1/NCNS, respectively, as well as Pt foil and PtO2reference at PtL3edge.iICP-OES results of M (Fe, Co, and Ni) metal loadings. It is worth noting that the EXAFS results perfectly match the DFT results (Supplementary Table 2 ). In summary, a close local structure of Co 1 Pt 1 /NCNS, Fe 1 Pt 1 /NCNS and Ni 1 Pt 1 /NCNS from simulated XANES and EXAFS fitting results strongly suggest the same deposition mechanism for Co, Fe, and Ni ALD on Pt 1 /NCNS, which indicates that this synthesis strategy can be a universal approach to achieve M 1 -pyrrolic N 4 type SACs using Pt 1 atoms. Table 1 Structural parameters of the M 1 Pt 1 /NCNS (M=Fe, Co, and Ni), foil, and oxide references extracted from quantitative EXAFS curve-fittings at Co, Fe, and Ni K edges. Full size table Theoretical understanding of deposition process Having resolved the structures of M 1 Pt 1 /NCNS and Pt 1 /NCNS, we carried out DFT calculations to elucidate the deposition mechanism. Considering the similar structure of Co, Fe, and Ni ALD precursors and local structures of Co 1 Pt 1 /NCNS, Fe 1 Pt 1 /NCNS, and Ni 1 Pt 1 /NCNS catalysts, typical Co ALD process is chosen for the following theoretical investigation. As revealed by the calculated Gibbs free energies shown in Fig. 5a , the Co(Cp) 2 has moderate adsorption (Δ G ad = −0.32 eV) but very high dissociation energy (Δ G de = 4.91 eV) on the pristine NCNS. Therefore, the physisorption of Co(Cp) 2 should be dominant on pristine NCNS. This physically and weakly adsorbed Co(Cp) 2 will lead to a low metal loading from inefficient deposition (Fig. 2i and Supplementary Fig. 5 ). Owing to the weak physisorption, Co species will easily aggregate because of the lack of strong chemical bonding with the substrate. Therefore, Co NPs were observed in the direct Co ALD process on NCNS (Fig. 1c ). However, when Pt 1 atoms are involved in the Co ALD process, the deposition model differs considerably. Although the adsorption of Co(Cp) 2 on Pt 1 atom is slightly weaker (Δ G ad = +0.06 eV), the dissociation energy of Co(Cp) 2 is reduced to Δ G de = 3.54 eV. The lower dissociation energy can be attributed to the electron transfer from the Cp ligand to the Pt 1 /NCNS, thus weakening the interactions between Co and Cp, which facilitates the dissociation process (Supplementary Fig. 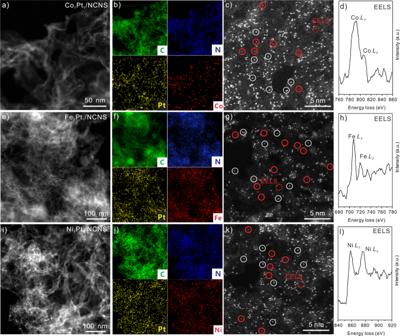Fig. 3: Morphology of M1Pt1/NCNS catalysts. HAADF-STEM images of Co1Pt1/NCNS (a), Fe1Pt1/NCNS (e), and Ni1Pt1/NCNS (i) at low resolution and corresponding EDX mapping (b,f, andj). HAADF-STEM images on Co1Pt1/NCNS (c), Fe1Pt1/NCNS (g), and Ni1Pt1/NCNS (k) samples. The white circles highlight the Pt single atoms. The red circles highlight the Co, Fe, and Ni single atoms, respectively.d,h, andlCorresponding EELS spectra at the location of red dash circle inc,g, andk. 19 and Supplementary Table 3 ). Considering it is a gas phase reaction, the Co(Cp) likely diffuses and deposits on the unoccupied pyrrolic N 4 sites through chemisorption. Such a strong chemical bonding of Co with pyrrolic N 4 sites will form a stable Co 1 structure after the O 2 pulse to remove the Cp ligand. It is worth noting that the introduction of O 2 may also remove the attached Cp ligand on the Pt 1 atom and recover the structure of Pt 1 /NCNS as shown in the Pt L 3 XANES and EXAFS results (Fig. 2g, h ). As a result, when the Co ALD is performed on Pt 1 /NCNS, Co single atoms will form and Pt 1 atoms will remain atomic dispersion (Fig. 5b ). The principle revealed by the theoretical calculation results indicates that this synthesis strategy could be universal for the rational design of SACs (Supplementary Fig. 20 ). Fig. 5: Illustration of theoretical understanding of the Co ALD process. a Theoretical reaction coordinate for Co(Cp) 2 deposition on pristine NCNS and Pt 1 /NCNS. The Gibbs free energies were calculated at T = 523 K and P = 1 atm. b Illustration of Co ALD process on Pt 1 /NCNS. The white, brown, blue, orange, and silver spheres represent H, C, N, Co, and Pt, respectively. Full size image Theoretical simulation and electrocatalytic performance of M 1 Pt 1 /NCNS The capability of application for the achieved M 1 Pt 1 /NCNS catalysts was further evaluated in electrochemical reactions. Prior to the experiment, we first studied the projected density of state (pDOS) of various M 1 -pyrrolic N 4 sites. As shown in Fig. 6a , the Co 1 -pyrrolic N 4 and Fe 1 -pyrrolic N 4 show higher DOS near the Fermi level than that of Ni 1 -pyrrolic N 4 . As is known, the high electron densities near the Fermi level could facilitate the adsorption of the proton (H + ) [41] , [42] , [43] . Further calculated hydrogen adsorption free energy on Co 1 -pyrrolic N 4 catalyst is closer to zero than that on Fe 1 -pyrrolic N 4 , indicating its relatively higher catalytic performance in HER (Supplementary Fig. 21 ). The Ni 1 -pyrrolic N 4 shows the weakest H adsorption ability, indicating its unsatisfactory HER activity. This theoretical prediction is confirmed by the experiment, in which the Co 1 Pt 1 /NCNS showed higher activity than Fe 1 Pt 1 /NCNS and Ni 1 Pt 1 /NCNS (Fig. 6b ). The higher catalytic activity of Co 1 Pt 1 /NCNS than the Pt 1 /NCNS could be attributed to the contributions of Co 1 atoms in HER (Supplementary Figs. 22 and 23 ) [44] , [45] , [46] . The Co 1 Pt 1 /NCNS also exhibits good stability without showing any obvious activity decrease after 8,000 cycles durability test (Supplementary Fig. 24 ). Although the Ni 1 -pyrrolic N 4 site exhibits low catalytic activity in HER, the high d -band center near the Fermi level on the Ni 1 atom (Fig. 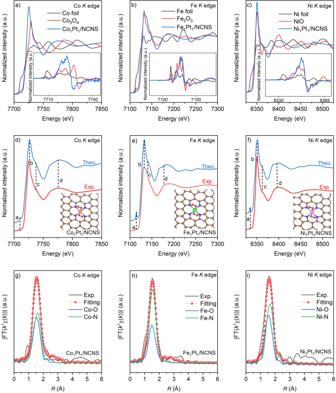Fig. 4: Identification of the local structure of M1Pt1/NCNS catalysts. a–cThe experimentalK-edge XANES spectra and first derivative curves (insets) of M1Pt1/NCNS and references samples.d–fComparison between the experimentalK-edge XANES spectra of M1Pt1/NCNS and the simulated spectra. Some of the main features reproduced are highlighted at points “a” to “d”. Fitting results of thek3-weighted FT spectrum of M1Pt1/NCNS at Co (g), Fe (h), and Ni (i) K edges. The white, brown, blue, red, orange, green, and pink spheres represent H, C, N, O, Co, Fe, and Ni, respectively. 6a and Supplementary Table 4 ) shows the promising application in OER [47] . In the experiment, the Ni 1 Pt 1 /NCNS shows the best catalytic performance among various SACs in OER (Fig. 6c ), which confirms the theoretical predication (Supplementary Figs. 25 and 26 ). The NCNS shows no catalytic activity in OER, indicating the carbon corrosion is not obvious (Supplementary Fig. 27 ). 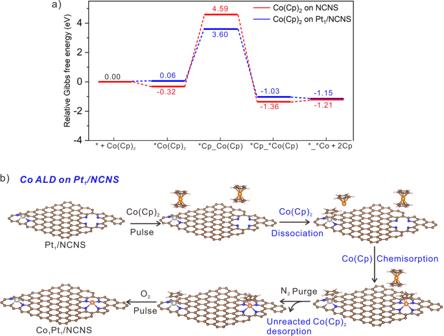Fig. 5: Illustration of theoretical understanding of the Co ALD process. aTheoretical reaction coordinate for Co(Cp)2deposition on pristine NCNS and Pt1/NCNS. The Gibbs free energies were calculated at T = 523 K and P = 1 atm.bIllustration of Co ALD process on Pt1/NCNS. The white, brown, blue, orange, and silver spheres represent H, C, N, Co, and Pt, respectively. 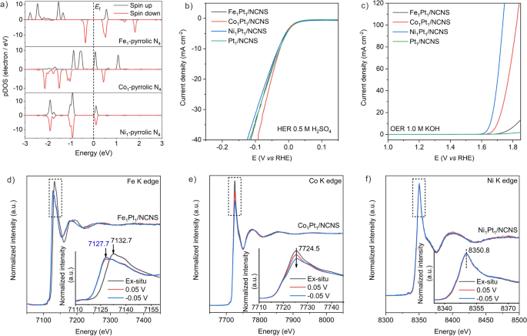Fig. 6: Theoretical and experimental electrocatalytic analysis on M1Pt1/NCNS (M=Co, Fe, and Ni). aProjected density of state (pDOS) on the M13dorbitals with the Fermi level set at zero. HER (b) and OER (c) LSV curves of M1Pt1/NCNS and Pt1/NCNS with IR correction.d–fOperandoXANES study on M1Pt1/NCNS catalysts in HER working conditions under different potentials at Fe, Co, and Ni K edges, respectively. Inserts: the enlarged area of XANES region in the dash square. Fig. 6: Theoretical and experimental electrocatalytic analysis on M 1 Pt 1 /NCNS (M=Co, Fe, and Ni). a Projected density of state (pDOS) on the M 1 3 d orbitals with the Fermi level set at zero. HER ( b ) and OER ( c ) LSV curves of M 1 Pt 1 /NCNS and Pt 1 /NCNS with IR correction. d – f Operando XANES study on M 1 Pt 1 /NCNS catalysts in HER working conditions under different potentials at Fe, Co, and Ni K edges, respectively. Inserts: the enlarged area of XANES region in the dash square. Full size image The non-noble SACs are reported to show promising HER performance but the nature of active sites under HER has not been systematically investigated yet. Therefore, in order to better understand the nature of single-atom sites under reaction, operando XAS experiments were conducted on M 1 Pt 1 /NCNS under HER at Fe, Co, and Ni K edges, respectively (Supplementary Fig. 28 ). As shown in Fig. 6d , a distinct energy chemical shift in the XANES white-line (WL) region can be observed on Fe 1 Pt 1 /NCNS at Fe K edge from 7132.7 to 7127.7 eV when the overpotential is applied on 0.05 V. This operando XANES results indicate the reduced oxidation state of Fe from +3 to +2. This Fe 3+ (d 5 )/Fe 2+ (d 6 ) redox transition is probably from the desorption of covered O species or impressed voltage, which would lead to a distorted Fe 2+ -N 4 structure [40] , [48] . As shown in Fig. 6e , an obvious WL intensity decrease can be found on the Co 1 Pt 1 /NCNS at Co K edge with the increasing overpotentials. Unlike the results of Fe (Supplementary Fig. 29a ), the E 0 on the Co K edge keeps constant (Supplementary Fig. 29b ). This decreased WL intensity indicates the filling of p electrons on Co, which could play an important role in the HER. The constant E 0 is likely from the charge redistribution from the hybridization among atomic orbitals in Co, which results in the negligible net effect on E 0 . In sharp contrast with the operando XANES results on Fe 1 and Co 1 atoms, neither the E 0 nor the WL intensity on Ni K edge of Ni 1 atoms showed obvious changes (Fig. 6f and Supplementary Fig. 29c ), indicating the Ni 1 -pyrrolic N 4 sites may be intact under HER. We also measured the operando XANES on the Fe, Co, and Ni -NPs/NCNS under HER for comparison, where no changes can be found on all the spectra (Supplementary Fig. 30 ). These apparently insensitive responses under electrochemical reactions might account for their poor activity in HER (Supplementary Fig. 31 ). For the first time, the synthesis of M 1 -pyrrolic N 4 type SACs has been successfully achieved using heterogeneously supported Pt 1 atoms as catalysts. This general M 1 -pyrrolic N 4 framework is confirmed by XANES simulation and EXAFS analysis. DFT calculations show that the Pt 1 atoms act as the catalyst to modulate the adsorption behavior and promote the dissociation of Co(Cp) 2 in Co ALD, which leads to the chemical binding of CoCp on the pyrrolic N 4 site and formation of Co single atoms. More importantly, this synthesis strategy can be extended to achieve Fe and Ni SACs. These SACs are evaluated under HER and the nature of single-atom sites are further unveiled by the operando XAS studies. In OER, the Ni 1 Pt 1 /NCNS catalyst show much better catalytic activity than the Fe and Co SACs counterparts, which is in excellent agreement with DFT prediction. These new findings extend the application fields of SACs to catalytic fabrication methodology, which is promising for the rational design of advanced SACs. The prominent covalent metal-support interaction bonding of M 1 atom (M=Fe, Co, Ni) with the local coordinated N-atoms provides a unique opportunity to further tune the catalytic properties through substrate design [49] , [50] . Synthesis of g-C 3 N 4 Twelve grams of urea was put into an alumina crucible with a cover and then heated to 580 °C at a rate of 3 °C/min in a muffle furnace and maintained at this temperature for 4 h. After cooling down to room temperature, ~600 mg of bulk g-C 3 N 4 was obtained. Synthesis of N-doped carbon nanosheet The synthesis method for the N-doped carbon nanosheets is based on a previous report [34] . Typically, 500 mg g-C 3 N 4 was mixed with 2.16 g glucose and dispersed in 40 mL of deionized water under sonication for 5 h. After that, the suspension was transferred to a Teflon autoclave and heated at 140 °C for 11 h in an oven. The product was collected by centrifugation and washed with water and ethanol several times, then dried under vacuum at 60 °C overnight. After that, the dried powder was heated up to 900 °C in Ar at a rate of 5 °C/min and maintained at this temperature for 1 h to achieve the N-doped carbon nanosheet (NCNS). Synthesis of Pt 1 /NCNS Pt was deposited on the as-prepared NCNS by ALD (Savannah 100, Cambridge Nanotechnology Inc., USA) using trimethyl(methylcyclopentadienyl)-platinum (IV) (MeCpPtMe 3 ) and O 2 as precursors. High-purity N 2 (99.9995%) was used as both a purging gas and carrier gas. The deposition temperature was kept at 150 °C, while the container for MeCpPtMe 3 was heated to 65 °C to provide a steady flux of Pt to the reactor. The manifold was kept at 115 °C to avoid any condensation [5] . The timing sequence of one cycle Pt ALD was 15s and 30s for MeCpPtMe 3 exposure and N 2 purge respectively. Subsequently, the ALD chamber was heated up to 250 °C, with 30s O 2 exposure and 30s N 2 purge to remove the ligand. Synthesis of M 1 Pt 1 /NCNS (M=Fe, Co, and Ni) The M ALD is conducted on the as-prepared Pt 1 /NCNS. The precursor used for Co, Fe and Ni are Ferrocene (Fe(Cp) 2 ), Cobaltocene (Co(Cp) 2 ) and Nickelocene (Ni(Cp) 2 ). High-purity N 2 (99.9995%) was used as both a purging gas and carrier gas. The deposition temperature was kept at 250 °C, while the container for M(Cp) 2 was heated to 90 °C to provide a steady flux of precursor to the reactor. The manifold was kept at 140 °C to avoid any condensation. The timing sequence of one cycle M ALD was 15s and 30s for M(Cp) 2 exposure and N 2 purge respectively. Subsequently, the ALD chamber was heated up to 300 °C, with 30s O 2 exposure and 30s N 2 purge to remove the ligand. Instrumentation TEM samples were prepared by drop-casting an ultrasonicated solution of dilute high-performance liquid chromatography grade methanol solution with the sample of interest onto a lacey carbon grid. The TEM characterization was carried out on a FEI Titan Cubed 80–300 kV microscope equipped with spherical aberration correctors (for probe and image forming lenses) at 200 kV. Atomic-resolution high-angle annular dark-field scanning transmission electron microscopy (HAADF-STEM) images were taken using a double spherical aberration-corrected FEI Themis microscope operated at 300 kV. The corresponding inner and outer collection semi-angles for HAADF imaging were 48–200 mrad. Dual EELS spectrum imaging was performed at a collection semi-angle of 28.7 mrad with a dispersion of 0.5 eV/channel. The metal loadings were analyzed using an inductively coupled plasma optical emission spectrometer (ICP-OES) with samples dissolved in hot fresh aqua regia overnight and filtered. Electrochemical measurements The electrochemical measurements were performed using a glassy carbon rotating-disk electrode (Pine Instruments) as the working electrode with carbon paper and a standard hydrogen electrode as the counter and reference electrodes, respectively. Ink for the electrochemical measurement was prepared by adding 2 mg of the catalyst into 1 mL ethanol, and Nafion (5% solution, Sigma-Aldrich, 20 μL), followed by sonication for 10 min. A working electrode was prepared by loading the ink (10 μL) on the glassy carbon electrode. The HER test was carried out in 0.5 M H 2 SO 4 with a scan rate of 0.01 V s −1 . The durability test was carried out in 0.5 M H 2 SO4 between −0.1 and 0.4  V at a scan rate of 0.1 V s −1 . The OER LSV polarization curves were measured in a O 2 -saturated electrolyte at a sweep rate of 5 mV s −1 . The durability test was carried out on a constant current density of 10 mA/cm 2 . The measured potential against the reference electrode was converted to a reversible hydrogen electrode (RHE). XAS measurements XAS measurements were conducted on the 061D superconducting wiggler at the hard X-ray microanalysis (HXMA) beamline at the Canadian Light Source (CLS) and beamline 20-ID-C at the CLS@APS of the Advanced Photon Source (APS), Argonne National Laboratory (ANL). At HXMA beamline, each spectrum was collected using fluorescence yield mode with a Canberra 32 element Ge detector. The beamline initial energy calibration for the different edges was made by using the corresponding metallic foils from Exafs Materials, and the same metallic foil was further set between two FMB Oxford ion chamber detectors downstream to the sample, making in-step energy calibration available for each individual XAFS scan. At 20-ID-C beamline, the XAS measurements were conducted at A Si (111) fixed-exit, double-crystal monochromator was used. Harmonic rejection was facilitated by detuning the beam intensity 15% at ∼ 1000 eV above the edge of interest. The measurements were performed in fluorescence mode using a four-element Vortex Si Drift detector. Details on the beamline optics and instruments can be found elsewhere [51] . Operando XAFS measurements were performed with catalyst-coated carbon paper using a custom-built cell. The carbon paper was pretreated with concentrated nitric acid at 80 °C overnight to ensure thorough electrolyte wetting. The catalyst ink was prepared with the same method as for the electrochemical measurements. The catalyst ink was dropped onto the carbon paper, and the backside of the carbon paper was taped with the Kapton film as the working electrode to ensure the entirety of the electrocatalyst had access to the H 2 SO 4 electrolyte. Carbon paper and Ag/AgCl were used as the counter and reference electrodes. To collect the XAFS spectra during the HER process, the cathodic voltages were held at constant potentials during the operando experiment from 0.05 to −0.05 V ( vs RHE), respectively. XANES modeling To further understand the nature of experimental resolved XANES features and address them to the structural and chemical nature of M (Fe, Co, and Ni) site occupancy and their corresponding local structural environment, DFT guided XANES theoretical modeling was carried out by using code FDMNES, following standard procedure [52] . For instance, a Co centered cluster was developed based on the structure model predicated by DFT optimized structures. The radius of the cluster is around 6 Å, corresponding roughly to the detection limit of the XAFS data. EXAFS data analysis The data reduction was using codes Athena [53] . The followed EXAFS R space curve fitting was performed using WINXAS version 2.3, following the procedure reported reference [54] . In brief, the first inflection point of the XANES edge was defined as the experimental E 0 , the post-absorption edge background was estimated and removed by cubic spline fits. Based on the local structural environment predicted by DFT theoretical modeling, the scattering amplitudes and phases were calculated using FEFF7.02 and further used for R space curve fitting [55] . The k rages for FT-EXAFS for Pt L 3 , Fe, Co, and Ni K edges are 3.15–11.57, 2.50–11.16, 2.37–10.90, and 2.33 to 10.48 Å −1 , respectively. Theoretical and computational methods First-principles DFT calculations were performed by using the spin-polarized Kohn–Sham formalism with the generalized gradient approximation (GGA) of Perdew-Burke-Ernzerhof (PBE) [56] , as implemented in the Vienna ab initio Simulation Package (VASP 5.4.4) [57] . The valence electronic states of all atoms were expanded in plane-wave basis sets with a cutoff energy of 400 eV, and gamma points were used for Brillouin zone integration. All atoms were allowed to relax until the forces fell below 0.02 eV Å −1 . The energy convergence criterion was set to 10 −5 eV. The zero-point vibrational energy (ZPE) and entropy corrections were performed by vibrational frequency analysis. We applied a graphene supercell with the surface periodicity of 8 × 8 including 128 atoms as a basis to construct the M-pyrrolic N 4 moieties. A vacuum region of 15 Å in the normal direction of the graphene plane was created to ensure negligible interaction between mirror images of the supercells.